Reactive nitrogen requirements to feed the world in 2050 and potential to mitigate nitrogen pollution Reactive nitrogen (Nr) is an indispensable nutrient for agricultural production and human alimentation. Simultaneously, agriculture is the largest contributor to Nr pollution, causing severe damages to human health and ecosystem services. The trade-off between food availability and Nr pollution can be attenuated by several key mitigation options, including Nr efficiency improvements in crop and animal production systems, food waste reduction in households and lower consumption of Nr-intensive animal products. However, their quantitative mitigation potential remains unclear, especially under the added pressure of population growth and changes in food consumption. Here we show by model simulations, that under baseline conditions, Nr pollution in 2050 can be expected to rise to 102–156% of the 2010 value. Only under ambitious mitigation, does pollution possibly decrease to 36–76% of the 2010 value. Air, water and atmospheric Nr pollution go far beyond critical environmental thresholds without mitigation actions. Even under ambitious mitigation, the risk remains that thresholds are exceeded. Globally, approximately 425 Tg of reactive nitrogen (Nr) is fixed every year from unreactive atmospheric dinitrogen (N 2 ) by natural processes in the oceans, on land and by human activity [1] . Nr is an important plant nutrient and about half of the globally fixed Nr fertilizes agricultural areas [1] . Agriculture thereby became the major driver of the global nitrogen cycle, in which total (terrestrial and oceanic) fixation doubled and terrestrial fixation more than quadrupled since the industrial revolution [1] , [2] . The nutrients reach the agricultural sector in the form of four major Nr sources: as inorganic fertilizers that were produced with the Haber–Bosch synthesis; as biologically fixed Nr, mainly driven by the cultivation of leguminous crops; through atmospheric deposition of Nr that previously volatilized elsewhere (about four-fifths stemming from anthropogenic sources [3] ); or through the release of organic Nr when soil organic matter depletes through soil management [4] . While passing through the agricultural supply chain, the Nr from these sources is subsequently lost on the field, in manure management, and as waste and sewage [1] , [5] , [6] , [7] , [8] . As there is little long-term storage of Nr in the agricultural sector, Nr sources correspond approximately to Nr losses, and are an easily communicable indicator for the disturbance of environmental systems by Nr pollution [9] , [10] . The subsequent destinies of lost Nr are diverse. Denitrification converts most of the Nr back into unreactive N 2 , but is also coupled to the production of the greenhouse gas and ozone-depleting substance N 2 O. If nitrogen is lost in reactive form through leaching or volatilization, it can cause a cascade of effects on the environment [7] , [11] . For instance, in combination with other nutrients, excessive Nr can lead to the disturbance of aquatic and terrestrial ecosystems through eutrophication. In the air, it leads to the formation of ozone and particulate matter. Negative impacts on human welfare [1] , [7] , [12] include direct health damages like cancer and asthma, as well as the loss of ecosystem services, affecting for instance the productivity of aquatic ecosystems and hence fishing [13] . In monetary terms, Nr pollution is estimated to cause damages in the magnitude of 0.3–3% of global gross domestic product (GDP) [1] . To reduce agricultural Nr pollution, a number of key mitigation actions are available for fertilization, livestock management, societal consumption and waste recycling [1] . However, it has not been quantitatively assessed by how much these mitigation measures could reduce Nr pollution at the global scale. Previous analysis of the global agricultural nitrogen cycle focussed mostly on the estimation of Nr flows in the present and past [14] , [15] , [16] , [17] , [18] as well as reference scenarios for future Nr flows and nitrogen fixation [4] , [19] , [20] , [21] , [22] . Quantitative estimates for Nr mitigation potentials are, so far, only based on simple calculations [1] , [10] , [23] or do not provide a comprehensive overview over the available mitigation measures and their interactions [15] , [22] , [23] . We apply a land-use and nitrogen-budget model [4] , [24] , [25] , [26] , [27] to analyse both reference and Nr mitigation scenarios for the global agricultural nitrogen cycle. Under different assumptions on consumption patterns and production technology, the model estimates the Nr sources required to satisfy a given future demand for agricultural products and assesses how the Nr is subsequently lost in the food supply chain. For a middle-of-the-road reference scenario, Nr sources can be expected to increase from currently 185 Tg Nr to 232 Tg Nr in 2050. Nr pollution will thereby further depart from environmental thresholds for air, water and atmospheric pollution. Subsequently, we analyse the following actions, which show substantial potential to mitigate Nr pollution: Reduced household food waste and recycling of food waste and sewage as fertilizers; lower share of animal-based calories in diets; efficient livestock management by improved feeding and higher recycling share for animal manure; and efficient fertilization of fields. The combined effect of all mitigation actions can lower Nr losses to 95 Tg Nr in 2050. The risk remains that this reduction is insufficient to bring Nr pollution below critical environmental thresholds. While leakage effects and externalities require a global approach to the regulation of Nr pollution, a spatial refinement of environmental thresholds is advisable for an efficient adaptation to Nr pollution. Reference scenario Our reference scenario without Nr mitigation is parameterized according to the ‘SSP2’ storyline of the shared socio-economic pathways [28] . This middle-of-the-road scenario assumes a world population of nine billion people in 2050 and a global GDP that more than triples to 230 trillion US Dollars at 2005 prices and adjusted for purchasing power parity (USD_05 PPP) [29] . Population groups which gain in prosperity demand a more affluent diet with a higher share of livestock products [30] . Therefore, crop production for food and feed increases by more than 50% compared with 2010, mainly by intensifying existing cropland. Over time, the developing countries adopt the industrialized livestock management of the Western regions. 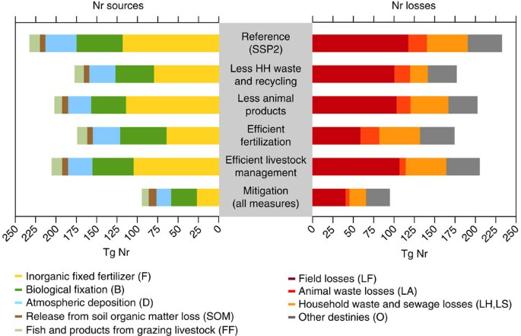Figure 1: Sources and losses of reactive nitrogen in the agricultural food supply chain in 2050. Units are in Teragram (Tg) reactive nitrogen (Nr). All scenarios are based on the storyline of the middle-of-the road scenario of the shared socio-economic pathways (SSP2), while they differ in respect to the implemented mitigation measures. Efficiency of Nr application on cropland improves in all world regions, but predominantly in the least efficient ones (Methods, Table 1 ). Table 1 Scenario parameters, entering the Model of Agricultural Production and its Impact on the Environment (MAgPIE) for the middle-of-the-road reference and mitigation scenario of the shared socio-economic pathways (SSPs). Full size table According to this reference scenario, Nr sources rise from 185 Tg Nr in the year 2010 to 232 Tg Nr in 2050 ( Fig. 1 ). This Nr stems mostly from inorganically fixed fertilizer (F) and biological fixation (B), and to a lesser extent from atmospheric deposition (D) and the release of Nr by the depletion of soil organic matter (SOM). Non-cropland-based Nr sources include fish and products from pasture-fed livestock (FF). While passing through the food supply chain, most of these nutrients are lost on the fields (LF), in household waste and sewage (LH, LS), and in animal waste management (LA). Other destinies (O) include post-harvest and processing losses, slaughter waste, the application of manure on pasture land and material use of agricultural products. Figure 1: Sources and losses of reactive nitrogen in the agricultural food supply chain in 2050. Units are in Teragram (Tg) reactive nitrogen (Nr). All scenarios are based on the storyline of the middle-of-the road scenario of the shared socio-economic pathways (SSP2), while they differ in respect to the implemented mitigation measures. Full size image Nr mitigation scenarios Subsequently, we estimate the effect of four Nr mitigation options on Nr sources and losses ( Fig. 1 ). The options were parameterized according to what is thought to be their maximum feasible potential (see Methods for details). They comprise the key mitigation actions proposed by the assessment ‘Our Nutrient World’ [1] for cropland production, the livestock sector, societal consumption and sewage. ‘Less household (HH) waste and recycling’ could lower Nr sources by 56 Tg Nr, removing the Nr losses that accrued in the production of wasted food, and recycling the nutrients from sewage and household waste to the fields. ‘Less consumption of animal products’ reduces Nr requirements by 30 Tg Nr, lowering losses in animal waste management as well as field losses by rendering parts of the feedstock production obsolete. ‘Efficient fertilization’ can reduce Nr losses on the field by 58 Tg Nr. ‘Efficient livestock management’ can lower required Nr sources by 27 Tg Nr through reduced losses in animal waste management and lower feedstock production. The combination of all mitigation measures fundamentally alters the flows in the nitrogen cycle by 2050 ( Fig. 2 ), and Nr losses are reduced to 95 Tg Nr. Crop biomass and grazed pasture are strongly reduced (C, P), and the dominant role of the livestock sector declines (A, P). Moreover, the absolute amount of recycled manure (RM) and crop residues (RR) as well as biological fixation (B) is reduced, but much less in relation to the savings of industrial fertilizer (F). The ‘full-chain efficiency’ [1] expressing the share of newly fixed Nr arriving at the consumer is increased to 69%, considerably higher than the current level (22%) as well as the level projected in SSP2 for 2050 (29%), and it exceeds even the proposed long-term target of 50% [1] . In total, the required Nr sources are reduced by 138 Tg. The reduction potentials of the individual mitigation actions are not independent, such that the combined reduction potential is lower than the sum of the individual reduction potentials. For example, reduced household waste diminishes the demand for agricultural products, resulting in lower down-stream field losses and thereby reducing the mitigation potential of more efficient fertilization. 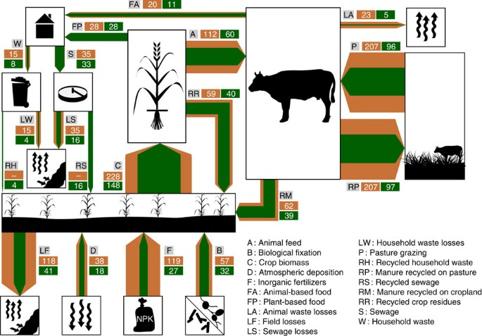Figure 2: Reactive nitrogen flows in agriculture in the year 2050. Units are in Teragram (Tg) reactive nitrogen (Nr). Arrows describe flows in the reference SSP2 scenario (brown) and after applying all Nr mitigation measures (green). Only major flows are presented in this figure, whileSupplementary Data 1gives an overview of all simulated flows. Figure 2: Reactive nitrogen flows in agriculture in the year 2050. Units are in Teragram (Tg) reactive nitrogen (Nr). Arrows describe flows in the reference SSP2 scenario (brown) and after applying all Nr mitigation measures (green). Only major flows are presented in this figure, while Supplementary Data 1 gives an overview of all simulated flows. Full size image Sensitivity analysis A sensitivity analysis, varying the major baseline and mitigation scenario parameters following the SSP 1 and 3 storylines shows that total Nr losses have an uncertainty range of at least 188–290 Tg Nr in the reference and 66–141 Tg Nr in the mitigation case. There are few additional mitigation options that are not covered by the analysed mitigation scenarios. These include lowering material use of agricultural products, abandoning the burning of crop residues or reducing and recycling processing waste (item O in Fig. 1 ). Our scenarios also did not consider morally problematic options like reducing population growth [31] , profound behavioural changes like diets solely based on leguminous proteins [32] or technological breakthroughs occurring before 2050 such as cereals that fix nitrogen [33] . Finally, the cultivation of bioenergy crops to replace fossil fuels or to sequester CO 2 was not considered in this study. Producing 100 Exajoule (one-fifth of current primary energy) of nutrient-efficient second generation bioenergy crops requires approximately 10 Tg of additional Nr sources, even under best practice conditions [25] . Upper estimates of monetized damage caused by current agricultural Nr pollution are as high as the agricultural value added [1] , [34] . As mitigation costs are by orders of magnitude lower than damage costs [35] , ambitious mitigation action can be well justified. However, cost-benefit analysis should be used with care as this tool aggregates preferences based on the willingness (and therefore ability) to pay. Given the highly unequal global distribution of wealth, this may lead to ambiguous outcomes, as it may for instance value overconsumption and ambitious environmental standards in rich countries higher than food security and a healthy environment in poor countries. To keep the Earth system within favourable conditions for human welfare, it was proposed to limit anthropogenic Nr fixation from all sectors below a ‘planetary boundary’ of 35 Tg Nr [9] , a value that would be far exceeded even with our mitigation scenarios. However, the height of this first and deliberately preliminary target was criticized to be arbitrary and unnecessarily low to avoid most pollution damage and also too low to provide food security [10] , [36] , [37] . A recent study [10] developed updated thresholds for air, water and atmospheric Nr pollution based on critical Nr concentrations (see Methods). Comparing Nr losses of agriculture with these critical thresholds ( Fig. 3 ) reveals that current pollution already exceeds all of these thresholds. Moreover, our results indicate in accordance with most other baseline scenarios [4] , [19] , [20] , [21] , [38] that Nr pollution will probably continue to rise and further depart from these thresholds [10] . 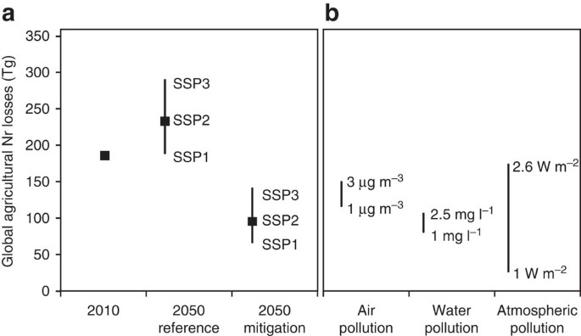Figure 3: Comparison of agricultural reactive nitrogen pollution with environmental thresholds. (a) global agricultural reactive nitrogen (Nr) losses in the year 2010 and in reference and mitigation scenarios for the year 2050. Scenarios are based on the storylines of the shared socio-economic pathways (SSPs). (b) environmental thresholds10for agricultural Nr losses are based on maximum ammonia (NH3) concentration (1–3 μg m−3) for air pollution, concentration of Nr in surface water (1 2.5 mg Nr l−1) for water pollution and nitrous oxide (N2O) emission trajectories leading to global warming targets (1–2.6 W m−2) for atmospheric pollution. Figure 3: Comparison of agricultural reactive nitrogen pollution with environmental thresholds. ( a ) global agricultural reactive nitrogen (Nr) losses in the year 2010 and in reference and mitigation scenarios for the year 2050. Scenarios are based on the storylines of the shared socio-economic pathways (SSPs). ( b ) environmental thresholds [10] for agricultural Nr losses are based on maximum ammonia (NH 3 ) concentration (1–3 μg m −3 ) for air pollution, concentration of Nr in surface water (1 2.5 mg Nr l −1 ) for water pollution and nitrous oxide (N 2 O) emission trajectories leading to global warming targets (1–2.6 W m −2 ) for atmospheric pollution. Full size image We show with this analysis that even under ambitious mitigation action, it remains uncertain whether water and atmospheric pollution can be reduced below the global critical thresholds in 2050, despite the substantial mitigation potential in crop farming, animal husbandry, food consumption and waste management. Due to the uncertainty of pollution projections and of appropriate thresholds, constellations are possible in which all respective thresholds are exceeded. Not represented in these ranges is the additional considerable uncertainty, which is connected to estimates of most Nr flows even for the current state [39] , in particular in regard to emissions [4] , [5] . Impacts of pollution are not linearly connected to the quantity of Nr losses, but are also determined by the distribution of Nr losses and vulnerable receptors in time, space and chemical form. Adapting to Nr pollution that cannot be mitigated is therefore the subsequent step to avoid damages, and possibly allows the loosening of environmental thresholds in places or times of low vulnerability. The above critical thresholds are therefore only a first step towards such a damage-minimizing distribution, and should be refined to a spatial and temporal explicit level. Still, the problem of Nr pollution has to be tackled with a global perspective. This is obvious for the greenhouse gas and ozone-depleting substance N 2 O, which disperses evenly in the atmosphere independent of the point of loss. But also for short-range pollutants, ambitious local environmental thresholds may lead to a shift of pollution sources to regions that fail to enforce environmental standards. Similarly, the required mitigation actions, like reducing food waste, do not only reduce local but also global environmental impacts. As these positive externalities cannot be fully internalized under uncoordinated local policies, global cooperation would be conducive when regulating Nr pollution. Land-use model The projections were made using the Model of Agricultural Production and its Impact on the Environment (MAgPIE) [4] , [24] , [25] , [26] , [27] , [30] , [40] , revision 7294. MAgPIE is a mathematical programming model that is used to create long-term scenarios and assessments of global land use. For a given food demand, the model estimates cost-optimal production patterns, and simulates major dynamics of the agricultural sector, like trade, technological progress and land allocation according to the scarcity of suitable land, water and economic resources [24] . As it treats agricultural products not only as economic values but also as physical goods, MAgPIE can perform analysis of material flows. The products in the model comprise 17 crop groups, each with individual above- and belowground crop residues, five livestock production types, eight types of conversion by-products originating from food processing, grazed pasture and scavenging. Products can be used for food, feed, other use (comprising material use and waste in the production chain) and seed, wherever applicable. Crop residues can be recycled to soils, burned in the fields, used as feed or used as material [4] . The demand for food enters the model as an exogenous trajectory [4] , [30] . Demand for material consumption and production waste is assumed to grow over time in proportion to food demand, while the demand for seed is a fixed share of crop production [4] . The demand for feed depends on the quantity of livestock production, as well as regional and livestock-specific feed baskets. In a first step, feed energy requirements per livestock product are calculated that entail the minimum requirements for maintenance, growth, lactation, reproduction and other basic biological functions of the animals. In addition, they comprise a general allowance for basic activity, temperature effects and expenditures for grazing. In a second step, these feed energy requirements are settled with regional livestock-specific feed baskets comprising concentrate feed, conversion by-products, crop residues and grazed biomass. As there are little data available on the amount of grazed biomass, grazed biomass was assumed to provide the remainder to fulfil the energy requirements of animals. The feed was distributed between the animal groups based on digestibility rules. Future developments within the livestock sector are implemented via convergence of the feeding systems to feed baskets that are parameterized according to the storyline, that is, a convergence to intensive European systems with high feed efficiencies and a higher share of concentrates [27] . The production of crops requires financial resources as well as land and water [41] . Cropland expansion leads to additional costs and is limited by biophysical conditions as well as by competing land-use activities. In additon to land expansion, the model can also invest into yield-increasing research and technology [42] . Crop growth functions connect crop harvest to the production of above- and belowground residues [4] . Similarly, the production of conversion by-products depends on fixed conversion factors multiplied with the regional crop supply [4] . Finally, livestock production requires financial resources, feed and water. To match global demand with supply, MAgPIE optimizes global land-use patterns and trade flows to minimize financial costs [24] . To account for trade restrictions and distortions, the socio-economic world regions have to produce a certain share of their internal demand [26] . The optimization problem is solved in consecutive time steps from 1995 to 2050, whereby the cropland area and the level of technology are passed on from one time step as input data to the consecutive time step [24] . Nr budget module MAgPIE was extended by a Nr flow module [4] that transforms all biomass flows in the model into Nr flows. The closed budget approach and a consistent connection of all Nr flows guarantee that the sum of Nr fixation, Nr release and inflows from other sectors corresponds to the sum of Nr losses and Nr flows to other sectors. Similarly, intermediary closed budgets are also used on a regional level for cropland soils, distribution and processing of agricultural products, livestock feeding, manure management and the household sector. While certain processes in MAgPIE such as crop production and water use are simulated spatially explicit on the level of clustered 0.5° grid cells, Nr flows and Nr budgets are calculated on the level of 10 world regions [4] . Nr in harvested crops (H), aboveground (RA) and belowground (RB) crop residues are estimated based on crop-specific crop growth functions and Nr contents of the individual plant components. The Nr derived from biological fixation within plants (B1) is estimated based on plant-specific shares of plant Nr derived from atmospheric fixation, while biological fixation by free-living microorganisms (B2) is estimated based on typical rates of Nr fixation per cultivated area. All belowground crop residues are assumed to be recycled to the field (RRB). In contrast, aboveground crop residues have to settle first the demand for feed from the livestock sector; moreover a fixed share of crop residues is assumed to be used for material purposes or is lost when residues are burned on the field. Only the remaining residues are recycled on fields (RRA). The Nr, which is released on croplands when soil organic matter depletes after the opening of new cropland (SOM), is calculated on the basis of model-endogenous land-use change activity, spatial-explicit carbon contents of natural soils, typical climate-specific shares of lost soil carbon under cropland management and a fixed carbon-to-nitrogen (C:N) ratio in soils. Atmospheric deposition (D) is estimated based on current deposition rates and is assumed to grow proportional to volatilized Nr losses. The Nr input of seeds (S) to cropland soils is based on regional plant-specific shares of the production that are used for seed [4] . To estimate the amount of manure recycled to croplands (RM), a budget approach is used. The Nr in animal feed (A) is estimated by assigning Nr contents to all feed items. The Nr in livestock products (FA) and slaughter waste (SW) is subtracted from the Nr in animal feed (A) to derive the amount of excreted Nr. While the feed from pasture is assumed to be excreted back on pasture land (RP1), other excrements are distributed between different animal waste management systems according to regional shares that change over time with scenario assumptions. Depending on their management, different shares of the nutrients are lost to volatilization and denitrification (LA); the remainder is recycled as organic fertilizers on cropland (RM) and pasture (RP2) [4] . For this study, the model was extended for a more detailed representation of food intake, food waste and sewage. Total food demand (intake+waste) and the share of animal-based products are estimated based on regression models [4] , [30] . The contribution of aquatic products to the protein supply by animal-based products is held constant at the value of year 2005 (ref. 43 ). To estimate household food waste, we assumed that the minimum waste share in all countries is 15%, accounting for inevitable losses and non-edible items like bones, kernel, husks and peels [44] . Moreover, we assumed based on plausible regional intake estimates for developed regions [45] that the per capita demand exceeding 2,200 kcal per capita per day is probably wasted. The resulting regional waste shares match well with current estimates [44] , but are dynamic for the future when per capita food demand rises. The Nr in sewage was estimated as the non-wasted share of food supply, not accounting for the relatively small share of Nr that is accumulated in human bodies or lost in sweat, hairs and nails [8] . Depending on the scenario assumptions, a share of sewage and organic waste is recycled to fields (RS, RW) or lost into the environment (LS, LW). Central to the model are regional nutrient budgets for cropland soils, which are used to determine the future requirements of fertilizers. Different Nr inputs to croplands have different fertilizer equivalents [1] , as they are to a different degree subject to losses on the field. Homogeneous Nr inputs (for example, industrial fertilizer) that can be easily distributed over the field have high equivalence values, while inhomogeneous Nr inputs (for example atmospheric deposition) have low equivalence values as their quantity, spatial distribution and timing cannot be controlled. Using a simplified approach, we distinguish only two categories in MAgPIE: First, Nr inputs from seed (S) and biological fixation within the plant (B1) are not taken up from the soil, and hence are not subject to losses by volatilization, leaching or denitrification. Nr from these inputs is therefore assumed to be fully incorporated into plant tissue. Second, we assume that all other Nr inputs are subject to losses before plant uptake and that only a share of the applied Nr inputs are withdrawn by the plant roots and incorporated into plant biomass. This share, named as soil Nr uptake efficiency (SNUPE), is a regional model parameter which reflects next to the climatic and biophysical conditions mostly the fertilization technology of farmers. As we do not consider the differences in fertilizer equivalences between individual soil Nr inputs like manure and inorganic fertilizers, a high value for SNUPE also implies that inhomogeneous fertilizers can be better integrated into crop fertilization, for example, by improved monitoring or by manure processing [1] . To calculate the application of inorganic fertilizers (F), we estimate the fertilization requirements to obtain a certain production under a given fertilization technology level. The Nr withdrawals from crop production (H+RA+RB) and the exogenous soil Nr uptake efficiency (SNUPE) determine the required Nr inputs from organic or inorganic fertilizers (equation (1)). Based on the availability of organic fertilizers, it is ultimately determined which amount of inorganic fertilizers is needed to balance out the budget [4] . The difference between inputs and withdrawals represents the field losses (LF) by denitrification, leaching and volatilization ( equation (2) ). A comprehensive overview over the estimates for the respective Nr flows can be found in the Supplementary Data 1 . Environmental thresholds The environmental thresholds for Nr pollution were adopted from a study [10] that estimates ‘planetary boundaries’ for Nr-related air, water and atmospheric pollution. For air pollution, a critical threshold was determined by limiting spatially explicit ammonia concentration to current levels; moreover concentration levels were capped where they exceed a maximum concentration (1–3 μg m −3 ). Likewise, water pollution was estimated based on maximum concentrations of Nr in surface water (1–2.5 mg Nr l −1 ). Critical thresholds for atmospheric pollution were estimated based on nitrous oxide (N 2 O) emission trajectories leading to global warming targets (1–2.6 W m −2 ). For each polluting Nr compound, the study [10] provides a risk indicator RI Ncompound =N Ncompound;critical /N Ncompound;present that indicates by how much the pollution N Ncompound;present in the year 2000 has to be reduced in order to reach the critical threshold N Ncompound;critical . Assuming that the ratio between N fixation and polluting compounds does not change, they multiply RI Ncompound by the agricultural nitrogen fixation of 121.5 Tg Nr in the year 2000 to derive thresholds for nitrogen fixation. However, total agricultural Nr losses is a more meaningful indicator for Nr pollution than total agricultural Nr fixation, as Nr losses also include Nr from sources like atmospheric deposition that may evolve disproportionally in the future. Therefore, to derive the thresholds for Nr losses presented in Fig. 3 , we multiplied their risk indicator RI Ncompound with our estimate for total Nr losses in the year 2000 (159 Tg Nr) instead of multiplying with total nitrogen fixation. The above critical thresholds are derived on the assumption that critical concentrations are not exceeded at any point of space. This assumption is not represented within MAgPIE, which calculates Nr flows only on the level of world regions. Especially on highly productive sites, thresholds are likely to be exceeded in our scenarios. Limiting production on these sites would lead to increased land expansion elsewhere with negative consequences on other environmental systems. Description of mitigation scenarios The scenario ‘Less household (HH) waste and recycling’ assumes a reduction of the waste share to 20%, resulting in a cut of per capita demand of each country to 2,750 kcal (2,200/0.8) in the year 2050. This is lower than the daily global per capita average in 2005 of 2,787 kcal, and considerably lower than the OECD average of 3,444 kcal [43] . Furthermore, we assume that half of the nutrients in household waste and sewage are recycled as fertilizers. The scenario ‘Less animal products’ assumes that no country derives more than 15% of its calories (29% of proteins) from animal-based products. This corresponds to a ‘demitarian’ western diet [1] , in which the share of animal-based calories is half of the current level in Western regions, and reverts the trend of the reference scenario ( Table 1 ). The scenario ‘Efficient fertilization’ estimates the effects of increasing SNUPE. High SNUPEs are difficult to reach, as this requires fertilizing the right amount of the right fertilizer at the right time and right place (4R), but also a better spatial integration of inhomogeneous Nr inputs like atmospheric deposition, manure and crop residues. We assume SNUPE increases globally from currently 53 to 75% in 2050 ( Table 1 ), approximately halving relative losses compared with today. A SNUPE of 75% is 15 percentage points higher than the value of the best-performing world region, Europe [4] , and also higher than the values in the most efficient agroecosystems [45] . The scenario ‘Efficient livestock management’ consists of two components. First, we assume that feed energy requirements of animals can be reduced by 25% relative to the reference scenario through better breeds and an improved deployment of existing feedstock. This increase in livestock productivity relative to the reference scenario corresponds well with the estimates of another study [46] if the trends are prolonged from 2030 to 2050. Lower feed intake also reduces manure excretion in the model. Second, the share of animal manure which is recycled from the stables to agricultural land is set to 90% in 2050, the highest plausible recycling share of the most efficient animal waste management systems [5] . The scenario ‘mitigation’ combines all above measures ( Table 1 ). For the sensitivity analysis, the parameterization of both reference and mitigation scenarios was adjusted to the SSP1 storyline with high potential for mitigation action, and to the SSP3 storyline with low mitigation potential. The adjusted parameters include population size, per capita demand, the share of food demand stemming from animal-based products, household waste and sewage recycling share, feed baskets and the recycling quota of manure. More information on the parameterization of the scenarios can be found in Table 1 and the Supplementary Data 2 . How to cite this article: Bodirsky, B. L. et al. Reactive nitrogen requirements to feed the world in 2050 and potential to mitigate nitrogen pollution. Nat. Commun. 5:3858 doi: 10.1038/ncomms4858 (2014).